An ecdysone-responsive nuclear receptor regulates circadian rhythms inDrosophila Little is known about molecular links between circadian clocks and steroid hormone signalling, although both are important for normal physiology. Here we report a circadian function for a nuclear receptor, ecdysone-induced protein 75 (Eip75/E75), which we identified through a gain-of-function screen for circadian genes in Drosophila melanogaster . Overexpression or knockdown of E75 in clock neurons disrupts rest:activity rhythms and dampens molecular oscillations. E75 represses expression of the gene encoding the transcriptional activator, CLOCK (CLK), and may also affect circadian output. PER inhibits the activity of E75 on the Clk promoter, thereby providing a mechanism for a previously proposed de-repressor effect of PER on Clk transcription. The ecdysone receptor is also expressed in central clock cells and manipulations of its expression produce effects similar to those of E75 on circadian rhythms. We find that E75 protects rhythms under stressful conditions, suggesting a function for steroid signalling in the maintenance of circadian rhythms in Drosophila . Timekeeping in Drosophila relies upon transcription-translation feedback loops, in which rhythmically expressed clock genes negatively regulate their own expression. In the major loop, the CLOCK-CYCLE (CLK-CYC) heterodimer activates transcription of the period ( per ) and timeless ( tim ) genes during the day, and in the middle of the night, the PER and TIM proteins heterodimerize and enter the nucleus to repress the activity of CLK-CYC [1] , [2] . In a second interlocked loop, CLK-CYC activate expression of the PAR Domain Protein 1 (Pdp1 ) ε and vrille (vri) genes, which encode an activator and a repressor, respectively, of the Clk gene. PDP1ε activates Clk transcription during the late night to early morning [2] , [3] . However, it is important to note that Clk mRNA levels are maintained at peak levels even in Clk Jrk and cyc 0 mutants that have very low PDP1, suggesting other transcriptional regulators of Clk expression [4] . In addition, structure-function analyses of the Clk promoter suggested that Clk expression can be regulated by transcription factors other than PDP1 and VRI [5] . Taken together, these studies implicate other transcription factors in Clk expression and possibly in the Drosophila molecular clock. The mammalian circadian clock is generated through similar mechanisms, whereby the negative regulators, CRYPTOCHROME (CRY) and PER, regulate the transcriptional activity of CLOCK and BMAL1 (mammalian orthologue of CYC) [6] . As in the Drosophila clock, the second loop is generated through autoregulation of one of the transcriptional activators, but in this case it is Bmal1 rather than Clock [7] . Nuclear receptors, REV-ERBα and β are transcriptional repressors of the Bmal1 gene [8] , [9] , whereas RORα is an activator [7] and both of these are targets of CLOCK-BMAL1. The closest Drosophila homologue of Rev-Erb is the nuclear receptor and ecdysone-induced protein, Eip75 (also known as E75) [9] , [10] . E75 mediates responses to ecdysone during development [11] and is also implicated in haem metabolism and signalling of gases such as carbon monoxide (CO) and nitric oxide (NO) [12] , [13] , [14] . However, although some components of the ecdysone signalling pathway are implicated in circadian rhythms [15] , it is not known if E75 has a role in the Drosophila circadian clock. In the present study, we identified E75 as a component of the Drosophila clock through an unbiased gain-of-function genetic screen for novel circadian genes. Overexpression as well as knockdown of E75 in clock neurons leads to arrhythmic or weak circadian behaviour. These manipulations also attenuate the molecular cycling of PER, indicating that they directly impact the molecular clock. We found that E75 acts as a repressor of Clk , and is itself subject to inhibition by PER. Thus, we have identified a mechanism for the previously proposed de-repressor function of PER on Clk expression [4] . Given the role of E75 in steroid signalling, which is involved in the response to stress, we also investigated its function under conditions of environmental stress. We found that expression of E75 protects the central clock against environmental stressors. E75 is a novel gene that regulates circadian rhythms As previously described [16] , we conducted a genetic screen for new circadian clock genes by overexpressing genes downstream of a randomly inserted EP (enhancer and promoter) element and assaying rest:activity rhythms. Of the 3,662 lines screened, one line (NE-30-49-10) contained an insertion in the promoter region of the E75 gene. This insertion lies upstream of all known isoforms of E75 , and its expression by the tim 27 -Gal4 driver (TG 27 ) increases expression of E75 approximately threefold in adult heads ( Supplementary Fig. 1a ). 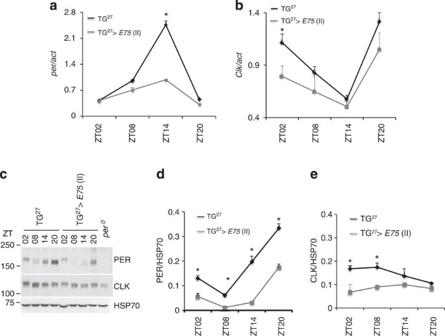Figure 1: Effect ofE75overexpression on the expression ofperandClkin adult heads. (a)permRNA expression in TG27controls and TG27>UAS-E75(II) flies during the indicated phases of an LD cycle. (b)ClkmRNA expression in TG27controls and TG27>UAS-E75(II) flies under LD cycle. (c) PER and CLK levels in the genotypes indicated above. A representative western blot is shown. PER and CLK levels are significantly lower in the TG27>UAS-E75(II) flies than in TG27control flies particularly at peak time points. HSP70 antibodies are used to control for loading. Quantification of four independent experiments shows significantly decreased (d) PER and (e) CLK levels in TG27>UAS-E75(II) flies relative to the TG27control flies. Asterisks above the bars denote significant differences between genotypes. *P<0.05 using unpaired Student’st-test. Error bars depict s.e.m. A molecular marker (Precision Plus Protein Dual Color Standards) was run to detect the exact molecular size of different proteins. This overexpression, which may be even greater in the targeted clock cells, rendered 96% of the flies arrhythmic under constant dark (DD) conditions ( Table 1A ; Supplementary Fig. 1b ). E75 is an ecdysone-induced protein and, as noted above, its closest homologue is REV-ERBα in mammals [17] . As TG 27 is expressed very broadly, we next overexpressed E75 under the control of the cry 24 - Gal4 and Pdf - Gal4 drivers, which are expressed at lower levels and also more specifically in clock cells. Pdf - Gal4 , in particular, is expressed only in the ventral lateral neurons, which are the central clock cells critical for behaviour in constant darkness. Overexpression of E75 by cry 24 - Gal4 resulted in loss of rhythms in 50% of the flies and those that were rhythmic, displayed significantly longer periods as well as weaker rhythms ( Table 1A ; Supplementary Fig. 1b ). Pdf - Gal4 -mediated E75 overexpression also produced a modest increase in period length and significantly reduced rhythm strength. In addition about 20% of the flies were arrhythmic under these conditions ( Table 1A ; Supplementary Fig. 1b ). Table 1 Circadian behaviour of flies with altered E75 expression levels under DD conditions. Full size table To verify that phenotypes obtained with the NE-30-49-10 insertion were due to overexpression of the E75 gene, we also overexpressed it using two independent UAS- E75 transgenes on the 2nd and 3rd chromosomes. E75 occurs as six different isoforms (see below), and we determined by sequencing that these transgenes overexpress the RC isoform. Overexpression of E75 by the TG 27 driver causes an approximately twofold increase in E75 mRNA levels ( Supplementary Fig. 1a ). The use of the TG 27 driver with either UAS- E75 transgene reduced the number of rhythmic flies. However, only TG 27 >UAS- E75 (II) flies showed a significant lengthening of period and decreased rhythm strength ( Table 1A ). On the other hand, Pdf - Gal4 -driven expression of UAS- E75 (III) rendered ~25% of the flies arrhythmic, although it did not produce a significant effect on other rhythm parameters. The weaker effect of the Pdf - Gal4 driver may be due to its restricted expression or to weaker strength. Regardless, these data support the idea that overexpression of E75 affects circadian behaviour. We next sought to determine whether loss of E75 impacts circadian rhythms. As null mutations of E75 are homozygous lethal, we used RNA interference (RNAi) to reduce the expression of E75 in clock cells, and analysed effects on circadian behaviour. We employed four independent lines carrying transgenic RNAi constructs targeted to the common region of E75 , two from the VDRC collection (GD and KK) and two from the Bloomington Stock Center (JF02257 and HMS01530). TG 27 -mediated knockdown of E75 levels led to ~75%, ~25% and ~42% arrhythmicity with JF, KK and GD RNAi lines, respectively, whereas knockdown via HMS RNAi was lethal ( Table 1B ). The GD RNAi lines showed a stronger effect on E75 transcript levels than KK lines ( Supplementary Fig. 1c ). Rhythmic flies for all three viable RNAi lines displayed significantly weaker rhythms and the JF line also yielded a significantly shorter period ( Table 1 ). Pdf - Gal4 -mediated E75 knockdown with the GD and JF RNAi lines also significantly reduced rhythmicity, but not circadian period ( Table 1B ). To improve the efficacy of knockdown, we co-expressed dicer2 with the RNAi constructs. Combining dicer2 with TG 27 caused lethality, so we coupled a slightly weaker tim driver, tim -UAS- Gal4 (TUG) and Pdf - Gal4 with dicer2 . TUG> dicer2 - or Pdf - Gal4 > dicer2 -mediated E75 knockdown led to a significant reduction in the number of rhythmic flies, and in most cases also in the strength of rhythmicity, with either the GD or JF RNAi transgene ( Table 1B ). To map the RNAi phenotype to E75 , we coupled the RNAi knockdown with genetic mutations of E75 . Although complete loss of E75 causes lethality, flies carrying one copy of the null allele (heterozygotes) survive and have normal rhythms ( Table 1B ). For instance, the E75 Δ51 strain contains an ~30 kb deletion that removes exons shared by all E75 isoforms [18] , and the heterozygotes display robust rhythms ( Table 1 ). However, restricted knockdown of E75 using Pdf - Gal4 in flies heterozygous for E75 Δ51 resulted in markedly fewer rhythmic flies than produced by Pdf-Gal4 in a wild-type background ( Table 1B ), indicating that the phenotype is attributable to loss of E75 function. As E75 manipulations had robust effects on circadian behaviour, we sought to determine if its expression was regulated in a circadian manner. E75 expresses six different mRNA isoforms (Flybase), three of which encode the same protein (RB, RE, RF). We designed PCR primers for the four that vary in protein sequence (RA, RB/E/F, RC, RD) and assayed expression at different times of day in adult brains. We detected moderate to robust cycling of four E75 isoforms in wild-type flies, with no cycling in the arrhythmic mutant Clk Jrk ( Supplementary Fig. 1d–g ), suggesting that expression of E75 is regulated by the circadian clock. In fact, a recent chromatin immunoprecipitation study indicated that CLK binds directly to the E75 promoter [19] . Alterations in levels of E75 affect the molecular clock To determine whether E75 affects molecular clock components, we first examined transcript levels of per and Clk in whole head extracts of flies overexpressing E75 (UAS- E75 II) via the TG 27 driver. Oscillations of per and Clk were dampened by E75 overexpression, in particular through a reduction in peak levels ( Fig. 1a,b ). We also measured PER and CLK protein levels through western blots of whole head lysates and found that these were significantly reduced in E75 overexpressing flies under light/dark (LD) conditions ( Fig. 1c–e ). Similar effects were observed under constant dark (DD) conditions; CLK expression was significantly reduced in flies overexpressing E75 as compared with the controls ( Supplementary Fig. 2a and b ). Figure 1: Effect of E75 overexpression on the expression of per and Clk in adult heads. ( a ) per mRNA expression in TG 27 controls and TG 27 >UAS- E75 (II) flies during the indicated phases of an LD cycle. ( b ) Clk mRNA expression in TG 27 controls and TG 27 >UAS- E75 (II) flies under LD cycle. ( c ) PER and CLK levels in the genotypes indicated above. A representative western blot is shown. PER and CLK levels are significantly lower in the TG 27 >UAS- E75 (II) flies than in TG 27 control flies particularly at peak time points. HSP70 antibodies are used to control for loading. Quantification of four independent experiments shows significantly decreased ( d ) PER and ( e ) CLK levels in TG 27 >UAS- E75 (II) flies relative to the TG 27 control flies. Asterisks above the bars denote significant differences between genotypes. * P <0.05 using unpaired Student’s t -test. Error bars depict s.e.m. A molecular marker (Precision Plus Protein Dual Color Standards) was run to detect the exact molecular size of different proteins. Full size image Next, we examined the effects of knocking down E75 using the same TG 27 driver to express UAS- E75 RNAi (GD) constructs. As shown in Table 1B , the GD line in particular led to a strong behavioural phenotype. As predicted by the overexpression data, per transcript levels were slightly, although not significantly, increased in flies in which E75 was knocked down, although PER protein levels were significantly different at ZT08 ( Fig. 2a,c,d ). Clk mRNA and protein levels were also significantly higher at specific times of day ( Fig. 2b,c,e ). Notably, under these conditions, per and Clk mRNA cycling did not appear to be affected ( Fig. 2a–e ). As with E75 overexpression, knockdown had robust effects on CLK expression under free-running conditions. CLK levels were significantly higher at CT08 and CT14 on the first day of DD in E75 knockdown flies ( Supplementary Fig. 2c and d ). 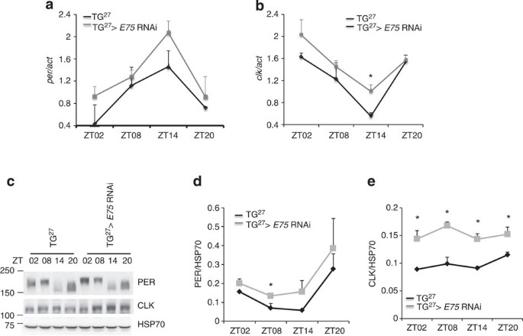Figure 2: Effects ofE75knockdown on the expression ofperandClkin adult heads. (a)permRNA expression in TG27controls and TG27>UAS-E75RNAi (GD) flies at the indicated time points of an LD cycle. (b)ClkmRNA expression in TG27controls and TG27>UAS-E75RNAi (GD) flies under LD cycle. (c) PER and CLK levels in the same genotypes as above. A representative western blot is shown. HSP70 antibodies are used to control for loading. Quantification of six independent experiments shows (d) PER and (e) CLK levels in TG27>UAS-E75RNAi (GD) flies and TG27control flies. Asterisks above the bars denote significant differences between genotypes. *P<0.05 using unpaired Student’st-test. Error bars depict s.e.m. A molecular marker (Precision Plus Protein Dual Color Standards) was run to detect the exact molecular size of different proteins. Figure 2: Effects of E75 knockdown on the expression of per and Clk in adult heads. ( a ) per mRNA expression in TG 27 controls and TG 27 >UAS- E75 RNAi (GD) flies at the indicated time points of an LD cycle. ( b ) Clk mRNA expression in TG 27 controls and TG 27 >UAS- E75 RNAi (GD) flies under LD cycle. ( c ) PER and CLK levels in the same genotypes as above. A representative western blot is shown. HSP70 antibodies are used to control for loading. Quantification of six independent experiments shows ( d ) PER and ( e ) CLK levels in TG 27 >UAS- E75 RNAi (GD) flies and TG 27 control flies. Asterisks above the bars denote significant differences between genotypes. * P <0.05 using unpaired Student’s t -test. Error bars depict s.e.m. A molecular marker (Precision Plus Protein Dual Color Standards) was run to detect the exact molecular size of different proteins. Full size image Clock proteins in adult head extracts are derived largely from the eyes, which do not contribute to the behavioural rhythm. Therefore, we also assayed PER levels through immunohistochemistry (IHC) in circadian behaviour-relevant brain clock neurons of flies with reduced levels of E75 . As the behavioural phenotype produced by E75 knockdown was somewhat variable (perhaps due to inefficient knockdown), we first selected arrhythmic flies by assaying their behaviour and then collected eight to ten flies from each experimental and control group at four different times of day. TG 27 -mediated knockdown of E75 resulted in dampened cycling of PER in constant darkness in different subsets of clock neurons ( Fig. 3a,b ). The dampening appeared to arise from significantly higher expression at trough time points (CT8 and CT14; Fig. 3a,b ). As the PDF cells are the ones most relevant for free-running behaviour, we quantified PER expression in these cells, and found significant differences at CT8 and 14 in the small LN v s and at CT8 in the large LN v s ( Fig. 3c,d ). PER cycling was also dampened under LD cycles; in fact, under these conditions, PER levels appeared to be relatively higher at all times in LN v s and LN d s of the E75 knockdown flies ( Supplementary Fig. 3a and b ). 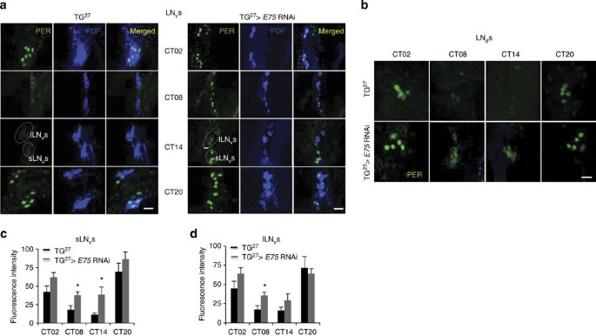Figure 3: Knockdown ofE75increases PER expression in brain clock cells. Flies from TG27and TG27>E75RNAi genotypes were tested for their circadian behaviour under DD conditions and on the 6th day 8–10 rhythmic TG27controls and 8–10 arrhythmicE75knockdown flies were used for IHC at each of the indicated time points. PER expression at different times of day in TG27>UAS-E75RNAi (GD) flies and TG27controls in the (a) small and large LNvs and (b) dorsal LNs (LNds). Quantification of PER staining from (c) sLNvs and (d) lLNvs subset of neurons in the TG27>UAS-E75RNAi (GD) flies (n=10) relative to TG27control flies (n=9). Asterisks above the bars denote significant differences between genotypes. *P<0.05 using unpaired Student’st-test. Error bars depict s.e.m. Time is indicated as CT (circadian time), where CT0 is 12 h after lights-off of the last LD cycle. Scale bar, 10 μm. Figure 3: Knockdown of E75 increases PER expression in brain clock cells. Flies from TG 27 and TG 27 > E75 RNAi genotypes were tested for their circadian behaviour under DD conditions and on the 6th day 8–10 rhythmic TG 27 controls and 8–10 arrhythmic E75 knockdown flies were used for IHC at each of the indicated time points. PER expression at different times of day in TG 27 >UAS- E75 RNAi (GD) flies and TG 27 controls in the ( a ) small and large LN v s and ( b ) dorsal LNs (LN d s). Quantification of PER staining from ( c ) sLN v s and ( d ) lLN v s subset of neurons in the TG 27 >UAS- E75 RNAi (GD) flies ( n =10) relative to TG 27 control flies ( n =9). Asterisks above the bars denote significant differences between genotypes. * P <0.05 using unpaired Student’s t -test. Error bars depict s.e.m. Time is indicated as CT (circadian time), where CT0 is 12 h after lights-off of the last LD cycle. Scale bar, 10 μm. Full size image We also assayed CLK levels of LN v s by IHC under LD cycles in TG 27 control and E75 knockdown flies. CLK expression was significantly, although modestly, higher at ZT01 in flies where E75 had been knocked down ( Supplementary Fig. 3c and d ). The small effect on CLK is consistent with the relatively minor shortening of circadian period in these flies ( Table 1 ). Although the effect on PER is greater, it is possible that the arrhythmic effects of E75 knockdown arise from effects on circadian output in addition to the molecular clock (see Discussion). E75 is a transcriptional repressor of the Clk gene The behavioural and molecular effects of E75 overexpression and knockdown strongly suggested an important role of this nuclear receptor in the molecular clock. To test for a possible function in the transcription of clock genes, we used cell culture assays. Given that the Drosophila E75 and mammalian REV-ERB proteins are so well conserved (~70%) in their DNA-binding domains ( Supplementary Fig. 4a ), we first tested E75 for effects on the native mouse Bmal1 promoter. We transfected Bmal1-luc ( Bmal1 promoter fused to luciferase) constructs into HEK293T cells and activated expression using mammalian RORα. Upon co-transfection with CMV- E75 , Bmal1-luc activity was significantly reduced approximately fourfold ( Supplementary Fig. 4b ). We then used a reporter construct for Clk in which the native promoter of Clk (~3.2 kb) was fused to a luciferase reporter gene [2] . The Clk promoter contains multiple PDP1/VRI and E75 sites, the latter based on their homology to target sites of mammalian REV-ERB proteins, which bind AGGTCA sites in A/T-rich regions [20] . We transfected the Clk-luc construct into HEK293T cells and assayed its expression in response to E75. As E75 is known to be a transcriptional repressor, but basal levels of Clk-luc are too low to detect further repression, we first activated expression of Clk-luc using PDP1 (pCDNA3-CMV- Pdp1ε ; Fig. 4a ). As reported previously [2] , we saw strong activation of the Clk promoter by PDP1ε in a dose-dependent manner ( Fig. 4a ). Next, we co-transfected these cells with different doses of E75 (driven by the CMV promoter in pCDNA3.1) and found that E75 strongly repressed Clk-luc activity ( Fig. 4a ). To verify that E75 acts on the Clk promoter, we constructed an E75-VP16 fusion protein, which is expected to turn E75 into an activator by introducing a VP16 activation domain, and tested its efficacy in regulating Clk-luc . We observed an increase of luciferase activity ( Supplementary Fig. 4c ), suggesting that E75 binds directly to the Clk promoter. 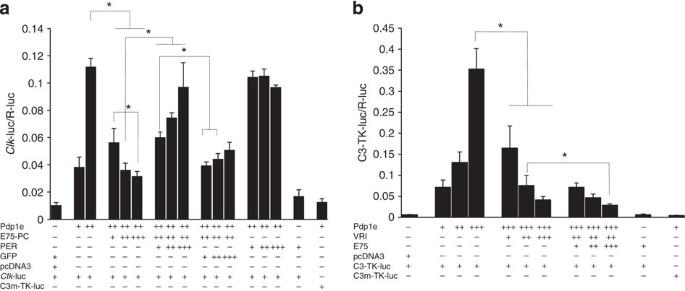Figure 4: E75 represses transcriptional activity of the nativeClkpromoter. (a) Mammalian HEK293T cells were transfected withClk-luc (50 ng) andrenilla-luc (10 ng) reporter (internal control) and with increasing doses of CMV-Pdp1ε(10 and 50 ng) or CMV-E75(50, 100 and 250 ng) and in some cases with CMV-per(10, 50, 100 ng). The +, ++ and +++ denote 10, 50 and 100 ng of DNA, respectively, except for the empty pCDNA3.1 vector. In addition, CMV-gfp(10, 50, 100 ng) was used as a control forper. The firefly luciferase activity was normalized torenilla-luc activity, and the fold induction (yaxis) was based upon comparisons with 10 ng of CMV expression vector alone transfections. Data represent an average of four experiments each performed in duplicate. Error bars depict standard error of the mean. C3m-TK-luc (a mutant promoter, which cannot be activated by PDP1) was used as an additional control. PDP1 ε and E75 significantly activated and repressedClk-luc, respectively, compared with empty vector pCDNA3.1 controls. PER significantly de-repressed the E75-mediated repression ofClkpromoter repression. (b) An artificial promoter, C3-TK-luc, was used instead of the nativeClk-luc promoter to determine if E75 acts as a co-repressor with VRI. C3-TK-luc contains three tandem consensus binding sites for PDP1/VRI but none for E75. Other details, including the dosage used, are same toa. PDP1 activates this promoter in a dose-dependent manner, and this is repressed by VRI. The highest dose of E75 enhances repression by VRI (*P<0.05. Two-way ANOVA, Tukey’s testpost-hoccomparison). Figure 4: E75 represses transcriptional activity of the native Clk promoter. ( a ) Mammalian HEK293T cells were transfected with Clk -luc (50 ng) and renilla -luc (10 ng) reporter (internal control) and with increasing doses of CMV- Pdp1ε (10 and 50 ng) or CMV- E75 (50, 100 and 250 ng) and in some cases with CMV- per (10, 50, 100 ng). The +, ++ and +++ denote 10, 50 and 100 ng of DNA, respectively, except for the empty pCDNA3.1 vector. In addition, CMV- gfp (10, 50, 100 ng) was used as a control for per . The firefly luciferase activity was normalized to renilla -luc activity, and the fold induction ( y axis) was based upon comparisons with 10 ng of CMV expression vector alone transfections. Data represent an average of four experiments each performed in duplicate. Error bars depict standard error of the mean. C3m-TK-luc (a mutant promoter, which cannot be activated by PDP1) was used as an additional control. PDP1 ε and E75 significantly activated and repressed Clk -luc, respectively, compared with empty vector pCDNA3.1 controls. PER significantly de-repressed the E75-mediated repression of Clk promoter repression. ( b ) An artificial promoter, C3-TK-luc, was used instead of the native Clk -luc promoter to determine if E75 acts as a co-repressor with VRI. C3-TK-luc contains three tandem consensus binding sites for PDP1/VRI but none for E75. Other details, including the dosage used, are same to a . PDP1 activates this promoter in a dose-dependent manner, and this is repressed by VRI. The highest dose of E75 enhances repression by VRI (* P <0.05. Two-way ANOVA, Tukey’s test post-hoc comparison). Full size image To determine if repression by E75 was specific to Clk , we transfected HEK293T cells with a per -luciferase reporter, in which luciferase is driven by a 4.6-kb fragment of the native per promoter that includes E box sites recognized by CLK [21] . As expected, the 4.6 per -luc reporter was activated by CLK; however, we failed to detect any repression by E75 ( Supplementary Fig. 4d ). On the other hand, PER significantly repressed its own transcription by inhibiting CLK-mediated per transcription ( Supplementary Fig. 4d ). These experiments strongly indicate specific repression by E75 at the Clk promoter. E75 affects transcriptional activity and levels of VRI Clk transcription is also known to be repressed by a well-known bZIP transcriptional factor, VRI, which directly competes with PDP1 to bind at the V/P box [2] . Interestingly, a genome-wide study aimed at identifying novel molecules induced by ecdysone signalling showed that vri expression was significantly increased [22] . In a separate study, vri expression was found elevated by ecdysone treatment in a tissue culture system [15] . As E75 expression is also induced by ecdysone signalling [10] , we examined whether E75 affects repression of Clk transcription by VRI. We used an artificial promoter containing three tandem consensus-binding sites for PDP1/VRI, but importantly lacking E75-binding sites, and co-expressed PDP1, VRI and E75. As expected, PDP1 activated Clk promoter-driven luciferase activity, whereas VRI repressed this activity in a dose-dependent manner ( Fig. 4b ). Interestingly, E75 further repressed expression of this promoter, suggesting that E75 modulates repression by VRI ( Fig. 4b ). To further address whether the two proteins act together to regulate transcription, we used a VRI-VP16 construct to directly activate the artificial Clk promoter, and found that the activation was potentiated by E75 ( Supplementary Fig. 5a ). As the experiments above utilized a Clk promoter that only contained sites for PDP1/VRI, we asked if direct binding of E75 to its own target sites on the Clk promoter could also modulate effects of VRI. 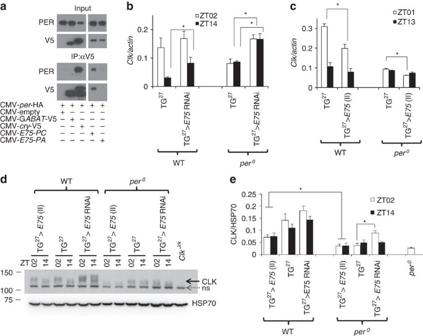Figure 5: PER interacts with E75 to de-repress expression of theClkpromoter. (a) Co-immunoprecipitation assay showed that PER physically interacts with E75. 100 ng of CMV-perHA was transfected with 200 ng of CMV-E75V5 (with two different isoforms RC and RA), CMV-cryV5, CMV-GABA-Transaminase(GABA-T) V5 and empty CMV vector. Anti-V5 antibody was used to pull down protein complexes. PER specifically binds with CRY but not with GABA-T, PER also binds strongly with E75-RC. The RA isoform was poorly expressed, hence weaker interaction with PER (lane 5 in IP: αV5). (b) Knockdown ofE75increasesClkmRNA expression in wild-type andper0flies. As inFig. 2,E75knock down by TG27significantly increasesClkmRNA levels in wild-type flies relative to TG27controls at ZT14. This effect is more striking inper0flies where baselineClkmRNA levels are quite low. (c) Overexpression ofE75reducesClkmRNA expression in wild-type andper0flies. As inFig. 1,E75overexpression by TG27significantly decreasesClkmRNA levels in wild-type andper0flies relative to TG27controls at ZT02. (d) CLK levels in TG27control, TG27>UAS-E75RNAi (GD) and TG27>UAS-E75(II) in wild-type andper0backgrounds are shown for two time points. HSP70 antibodies are used to control for loading. Molecular marker (Precision Plus Protein Dual Color Standards) was run to facilitate detection of different proteins. ns, non-specific. (e) Quantification of four independent western blots is shown. Asterisks above the bars denote significant differences between genotypes. *P<0.05 using unpaired Student’st-test. Error bars depict s.e.m. Thus, we used a native Clk promoter, and found that E75 significantly reduced VRI-VP16-mediated activation of Clk ( Supplementary Figure 5b ). These data indicate that E75 can repress Clk directly, but probably also affects VRI repression of the Clk promoter. As vri expression is increased by ecdysone signalling [15] , [22] , we also examined whether E75 affects VRI levels. Knocking down E75 levels in clock cells significantly reduced VRI levels and overexpression slightly elevated trough levels of VRI, indicating that E75 interacts with VRI on multiple levels ( Supplementary Fig. 5c,d ). PER interacts with E75 and acts as a de-repressor for Clk transcription Low levels of Clk mRNA in mutants lacking PER ( per 01 ) are thought to reflect a de-repressor function of PER, in other words suggesting that PER suppresses activity of some repressor [4] . However, PER is not known to affect VRI-dependent repression of Clk , as the effect of VRI on Clk expression is similar in wild-type and per null backgrounds [2] . Because E75 had robust effects on Clk transcription in cell culture assays, we asked if PER affects repression of Clk by E75. To address this question, we used the same luciferase-based transcription assays in cell culture. As above, the native Clk-luc promoter was activated by PDP1ε and repressed by E75, and subsequently PER (driven by the CMV promoter) was added in a dose-dependent manner. Interestingly, PER strongly inhibited repression of Clk by E75, suggesting that it acts as a de-repressor ( Fig. 4a ). A construct expressing GFP did not affect repression by E75, demonstrating that the de-repression did not result merely from the presence of another transfected protein ( Fig. 4a ). In the absence of E75, PER did not affect transcriptional activity of the Clk promoter, supporting the idea that it acts as a de-repressor rather than a co-activator ( Fig. 4a ). To determine whether E75 and PER physically interact, we co-transfected them into mammalian HEK293T cells as well as into Drosophila S2 cells and conducted co-immunoprecipitation assays. E75 tagged with V5 pulled down PER in HEK293T cells ( Fig. 5a and Supplementary Fig. 6a ). CRY-V5 also pulled down PER under these conditions, whereas a nonspecific GABA-T-V5 (GABA-transaminase fused to a V5 tag) protein did not, indicating specificity of the interaction between E75 and PER and also between CRY and PER ( Fig. 5a and Supplementary Fig. 6a ). Similar results were obtained in Drosophila S2 cells, where PER pulled down V5-tagged E75 ( Supplementary Fig. 6b ). Figure 5: PER interacts with E75 to de-repress expression of the Clk promoter. ( a ) Co-immunoprecipitation assay showed that PER physically interacts with E75. 100 ng of CMV- per HA was transfected with 200 ng of CMV- E75 V5 (with two different isoforms RC and RA), CMV- cry V5, CMV- GABA-Transaminase (GABA-T) V5 and empty CMV vector. Anti-V5 antibody was used to pull down protein complexes. PER specifically binds with CRY but not with GABA-T, PER also binds strongly with E75-RC. The RA isoform was poorly expressed, hence weaker interaction with PER (lane 5 in IP: αV5). ( b ) Knockdown of E75 increases Clk mRNA expression in wild-type and per 0 flies. As in Fig. 2 , E75 knock down by TG 27 significantly increases Clk mRNA levels in wild-type flies relative to TG 27 controls at ZT14. This effect is more striking in per 0 flies where baseline Clk mRNA levels are quite low. ( c ) Overexpression of E75 reduces Clk mRNA expression in wild-type and per 0 flies. As in Fig. 1 , E75 overexpression by TG 27 significantly decreases Clk mRNA levels in wild-type and per 0 flies relative to TG 27 controls at ZT02. ( d ) CLK levels in TG 27 control, TG 27 >UAS- E75 RNAi (GD) and TG 27 >UAS- E75 (II) in wild-type and per 0 backgrounds are shown for two time points. HSP70 antibodies are used to control for loading. Molecular marker (Precision Plus Protein Dual Color Standards) was run to facilitate detection of different proteins. ns, non-specific. ( e ) Quantification of four independent western blots is shown. Asterisks above the bars denote significant differences between genotypes. * P <0.05 using unpaired Student’s t -test. Error bars depict s.e.m. Full size image We next determined whether PER contributes to the regulation of Clk via E75 in vivo . Thus, we examined Clk mRNA levels in response to manipulations of E75 in the presence and absence of PER. As reported earlier, we found that per 0 flies express relatively low levels of Clk mRNA [4] ( Fig. 5b,c ). Knockdown of E75 in a per 0 background increased Clk mRNA to peak levels in wild type, supporting the idea that E75 keeps Clk mRNA low in per 0 flies ( Fig. 5b ). In wild-type flies, the effect of E75 knockdown on Clk mRNA was restricted to the trough time point and was less than in per 0 , perhaps because E75 has limited contribution to Clk expression in the presence of the de-repressor PER. We also assayed Clk mRNA levels in wild-type and per 0 backgrounds under conditions where E75 was overexpressed with the TG 27 driver. As noted in Fig. 2 , overexpression of E75 reduced Clk mRNA in wild-type flies. In per 0 flies also, overexpression of E75 reduced the expression of Clk mRNA, although the difference was small, perhaps because Clk levels were already low ( Fig. 5c ). The effect of knockdown and overexpression of E75 on Clk mRNA levels in a per 0 background indicate that endogenous PER affects E75 action at the Clk promoter. To further analyse the genetic interaction between PER and E75, we also compared CLK protein levels in wild-type and per 0 genetic backgrounds, following overexpression or knockdown of E75 . Knockdown of E75 increased CLK protein in wild-type and per 0 flies, but in these experiments the difference was significant only in per 0 (note that there is variability in the effect on CLK), again supporting the idea that E75 contributes more to CLK expression in per 0 flies. However, the increase in the protein was not as great as in the mRNA, suggesting that other factors keep CLK low in per 0 flies. Overexpression of E75 resulted in a greater overall reduction of CLK in a per 0 background than in wild type, again most likely because CLK levels are already low in per 0 ( Fig. 5d,e ). Ecdysone signalling regulates circadian behaviour Previous studies have reported that steroid hormone signalling induces E75 expression to regulate critical developmental processes [23] , [24] . However, ecdysone signalling is also present in adult stages, and mutations that alter hormone or receptor levels affect diverse processes such as behaviour, stress resistance, reproduction and lifespan [11] . In fact, disruption of ecdysone signalling has been associated with alterations in circadian behaviour and in sleep [15] , [25] . Therefore, we assayed effects of manipulating ecdysone signalling specifically in clock neurons on rest:activity rhythms and on the molecular clock. We first established that the ecdysone receptor (EcR) is expressed in circadian neurons. EcR has three isoforms A, B1 and B2, which differ in their N termini [26] . We obtained antibodies to EcR isoforms and verified that they recognize these specific proteins, based on their reduced levels in EcR RNAi lines and increased levels in flies that overexpress EcR (data not shown). The EcR-A antibody is specific for EcR-A isoform, and the EcR-C antibody is known to detect all three isoforms of EcR [27] . Through IHC experiments, we identified distinct expression of the EcR-A-specific isoform and perhaps other isoforms (as detected by EcR-C) in adult LN v s as well as in the 3rd instar larval stage ( Fig. 6a,b ). To alter EcR activity in clock cells, we utilized RNAi, dominant negative and overexpression approaches, as null mutations of EcR are lethal. The dominant negative form of EcR (EcR Δ ) cannot be activated by ecdysone and interferes with the activity of endogenous EcR, leading to deficiencies in EcR function [26] . Expression of EcR-B1 Δ by Pdf - Gal4 resulted in a significant increase in period and decreased rhythm strength ( Table 2A ). Using TUG, UAS-EcR-B1 Δ was expressed in broader sets of clock cells, and resulted in a much longer period (~26 h) and ~30% arrhythmicity, but surprisingly less of an effect on the strength of rhythms in rhythmic flies ( Table 2A ). We also expressed EcR-B1 Δ using the even stronger clock cell Gal4 (TG 27 ), which resulted in 100% lethality. As reported by Itoh et al . [15] , knockdown of EcR using RNAi also yielded circadian phenotypes. EcR-A RNAi in PDF-positive cells did not alter period but significantly reduced rhythm strength ( Table 2A ). On the other hand, EcR-A RNAi using the TUG driver led to a significantly longer period ( Table 2A ), although again, with less of an effect on rhythm strength. 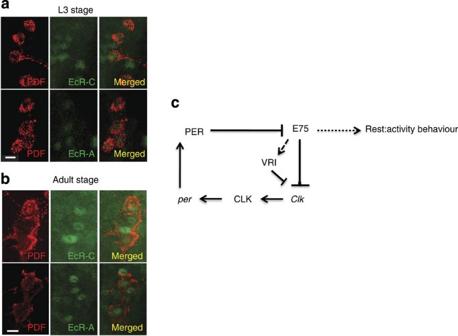Figure 6: Incorporating EcR and E75 in the molecular clock. EcR is expressed in clock cells of larval (a) and adult brains (b). EcR is detected with two different mouse anti-EcR antibodies (EcR-A and EcR-C) and PDF is stained with a rabbit anti-PDF antibody. EcR-C antibody detects all isoforms of EcR (A, B1 and B2), whereas EcR-A detects the RA-specific isoform of EcR. Scale bar, 10 μm. (c) Model for the role of E75 in theDrosophilamolecular clock. E75 repressesClktranscription, and this repression is inhibited by PER, which thus acts as a de-repressor ofClk. PER can also modulateClkexpression through VRI (as VRI is a transcriptional target of CLK, which is regulated by PER), but this is not shown here for the sake of simplicity. In addition, E75 also regulates VRI expression in such a way that overexpression or knockdown of E75 increases or reduces the VRI levels, respectively, thus indirectly affecting the CLK expression. Under stressed (nutritional and temperature) conditions, E75 is required to maintain robust rhythms. Figure 6: Incorporating EcR and E75 in the molecular clock. EcR is expressed in clock cells of larval ( a ) and adult brains ( b ). EcR is detected with two different mouse anti-EcR antibodies (EcR-A and EcR-C) and PDF is stained with a rabbit anti-PDF antibody. EcR-C antibody detects all isoforms of EcR (A, B1 and B2), whereas EcR-A detects the RA-specific isoform of EcR. Scale bar, 10 μm. ( c ) Model for the role of E75 in the Drosophila molecular clock. E75 represses Clk transcription, and this repression is inhibited by PER, which thus acts as a de-repressor of Clk . PER can also modulate Clk expression through VRI (as VRI is a transcriptional target of CLK, which is regulated by PER), but this is not shown here for the sake of simplicity. In addition, E75 also regulates VRI expression in such a way that overexpression or knockdown of E75 increases or reduces the VRI levels, respectively, thus indirectly affecting the CLK expression. Under stressed (nutritional and temperature) conditions, E75 is required to maintain robust rhythms. Full size image Table 2 Circadian behaviour of flies with altered EcR expression levels under DD conditions. Full size table We also overexpressed different isoforms of the EcR gene using Pdf - Gal4 and TG 27 drivers. Pdf - Gal4 -mediated overexpression of the different isoforms produced phenotypes of varying strength, with two isoforms (A and B2) reducing rhythm strength and one (A) also reducing the number of rhythmic flies ( Table 2B ). TG 27 -mediated overexpression of EcR-A , B2 and C, which expresses a common region from all three isoforms of EcR , that is, A, B1 and B2 (ref. 26 ), resulted in phenotypes that included significantly longer periods, reduced rhythm strength and increased arrhythmia ( Table 2B ). However, the effects varied somewhat from one isoform to the other ( Table 2B ). EcR is a well-known transcription factor regulating E75 levels, and so it likely contributes to E75 expression in clock cells [28] . We assayed the levels of different isoforms of E75 in the brains of flies where EcR-B1 levels were knocked down. Consistent with previous findings, we found that E75-RA, RB and RC isoforms were reduced by knockdown of EcR ( Supplementary Fig. 7a ). EcR knockdown also increased CLK expression, although the effects were milder than seen with E75 reduction ( Supplementary Fig. 7b and c ), perhaps because EcR can affect Clk in multiple ways through different signals [15] . These data indicate though that effects of EcR, like those of E75, are not going solely through the molecular clock (see Discussion). E75 protects the central clock under conditions of stress In adults, ecdysone signalling is increased upon exposure to stressful environments [25] , [29] . As E75 is a direct target of EcR, we asked if signalling through E75 is important in the presence of environmental stressors. To test this idea, we subjected adult flies to two different stressful conditions that are known to increase ecdysone signalling: low nutrition and high temperature [30] , [31] . For nutritional stress, we varied the amount of sucrose (1, 2 and 5%) in the 2% agar medium (see Methods for details), whereas for temperature stress, we tested temperatures of 25 (regular), 28 and 32 °C. Control flies (iso31 or UAS/Gal4 alone) did not show changes in circadian period upon temperature or nutritional stress ( Table 3 and Supplementary Table 1 ) and for the most part they remained rhythmic, although the lines carrying the drivers alone showed some loss of rhythm. Environmental stressors (temperature and nutritional) produced a much stronger effect when E75 was knocked down in all clock neurons (TUG> E75 RNAi), with flies displaying increased arrhythmia ( Table 3B and Supplementary Table 1 ). Notably, the period of the rhythmic flies did not change significantly even with E75 knocked down ( Table 3B and Supplementary Table 1 ). We also used Pdf - Gal4 ; dicer2 to knock down E75 levels under these two conditions, and observed a significant decrease in fast Fourier transform (FFT) values (that is, rhythm strength) and number of rhythmic flies ( Table 3B and Supplementary Table 1 ). Table 3 Circadian behaviour of flies with low E75 under nutritional stress conditions. Full size table To exclude the possibility that any manipulation of the clock renders it more sensitive to environmental stressors, we subjected a Clk allele, Clk hypo , which has dampened molecular oscillations and a long period (~26.5 h; unpublished observations; see Methods for details regarding the lesion), to the same stress conditions. Approximately 60–70% of the Clk hypo flies remained rhythmic under low-nutrient or high-temperature conditions ( Supplementary Table 2 ). Thus, the effect of the stressors was specific for flies that had low levels of E75. To test whether EcR also impacts the circadian clock under stressful conditions, we assayed locomotor activity rhythms of flies in which EcR had been knocked down under high-temperature conditions. As with E75 knockdown, a reduction in EcR levels (A and B1 isoforms) in clock cells led to weakened rhythm strength as well as increased arrhythmicity under conditions of stress ( Supplementary Table 3 ). Importantly, control flies and flies with reduced E75 had similar responses to stress in terms of locomotor activity levels, lifespan and food intake ( Supplementary Fig. 8 ). Taken together, these data suggest that ecdysone signalling promotes maintenance of rhythms under stressful conditions without significantly affecting daily activity levels, food consumption and longevity. We report here that E75, a nuclear hormone receptor induced by ecdysone signalling in Drosophila , regulates circadian behaviour. This finding was based upon an unbiased, forward genetic screen, in which E75 stood out as a robust modulator of behavioural rhythms. Although the focus of this study is on rest:activity rhythms, which are controlled by the central clock in the brain, the western blot data suggest that E75 is also a component of peripheral clocks in the head. It is likely that not just E75, but ecdysone signalling in general impacts peripheral circadian function. We have also identified a molecular mechanism by which E75 affects the clock. Finally, we show that, in addition to its role in the clock under normal conditions, E75 protects the clock in times of stress. The latter may be related to its function in a steroid signalling pathway. In vertebrates, the closest homologues of E75 are members of the REV-ERB family. Although REV-ERB is a part of the mammalian clock mechanism, the Drosophila orthologue, that is, E75, was previously not known to have a circadian function. Here we show that E75 is an inhibitor of Clk transcription, by itself and also in conjunction with VRI. Before this work, it was thought that the role of nuclear hormone receptors in mammalian clocks was served by PAR domain containing proteins, PDP1 and VRI, in Drosophila [2] . Thus, although REV-ERB and ROR regulate expression of Bmal1 in mammals, PDP and VRI regulate expression of the other transcriptional activator, Clk , in flies. Our data indicate that E75 does indeed function in the Drosophila clock, much as its mammalian counterpart does ( Fig. 6c ). One may ask why E75 is required if the second feedback loop is maintained by PDP1 and VRI. We suggest that E75 couples the clock to extracellular cues. Induction of E75 by the steroid hormone, ecdysone, likely allows the clock to respond to endocrine signals and perhaps other ligands (further discussed below). As reported here, E75 signalling may be particularly relevant under conditions of stress. Tissue culture experiments do not indicate a direct effect of E75 on per expression, although we cannot exclude the possibility that it does so in flies, as suggested by the robust effect of E75 overexpression on per mRNA and protein levels ( Fig. 1 ). However, E75 interacts with PER to regulate transcription of Clk . Indeed, this work reveals a new role for Drosophila PER as a de-repressor. As noted above, earlier studies showed that PER promotes expression of Clk , but the underlying mechanisms were not identified. We find that it does so by reducing the inhibitory effect of E75 on CLK. It may do so by affecting DNA binding of E75 or perhaps even by destabilizing it. Regardless, these data are reminiscent of mammalian PER, which acts as a de-repressor with some nuclear receptors and a co-activator with others [32] . Indeed, mammalian PER2 and REV-ERB-α physically interact [32] , [33] , as we show here for PER and E75. We suggest that crosstalk between components of the two loops is a conserved mechanism that serves to maintain a robust cycle. On the one hand, Drosophila PER inhibits activity of the CLK/CYC complex to generate a negative feedback loop; meanwhile, it interacts with nuclear hormone receptors like E75 to promote Clk gene expression in the positive feedback loop. Although this study only examined effects of PER on E75-mediated repression of CLK, it is likely that there are other circadian targets of E75 that are modulated by PER. Future studies should help to clarify the extent to which E75 impacts transcription within the circadian network. Importantly, the data on E75 presented here provide insight into some of the unresolved questions in the clock field—for instance, why Clk mRNA levels are low in per 0 flies. Although E75 appears to act as a component of the molecular clock, its effects on behaviour are probably not going entirely through the clock. Knockdown of E75 increases Clk , which typically shortens period [34] , but does not cause arrhythmia. Along the same lines, per rhythms dampen, but are not eliminated upon E75 knockdown, and this dampening is not expected to render flies arrhythmic. We suggest that effects of E75 on circadian period are mediated by Clk , but in addition E75 affects circadian output, which contributes to the arrhythmia caused by knockdown. As mentioned above, E75 may affect the transcription of other genes, perhaps even in a circadian manner. We suggest that E75 is regulated by the clock, which is supported by experiments showing direct binding of CLK to the E75 promoter [19] . Although this is the first report of an ecdysone-induced nuclear receptor in the Drosophila central clock mechanism, ecdysone signalling has been previously linked to circadian function. Early gene at 23 ( E23 ), which suppresses the response to ecdysone, is required for normal circadian rhythms in Drosophila [15] . E23 encodes a membrane-bound ATP-binding cassette (ABC) transporter that is induced by ecdysone in central clock neurons, and its knockdown in these neurons (LN v s) increases expression of the clock gene, vrille , and lengthens circadian period [15] . The relationship between E75 and E23 is not known; it is possible that ecdysone signalling activates both molecules, which then have independent effects on the clock. Alternatively, effects of E75 (overexpression and knockdown) on VRI expression as well as cell culture data indicate that E75 may also regulate VRI to modulate Clk expression and circadian behaviour. Importantly, disruption of EcR signalling also affects rhythms. Loss of EcR can have developmental effects on clock cells [35] , but we note that many of our manipulations of EcR change circadian period without causing arrhythmia, indicating a more specific effect on clock function. Both EcR and E75 are required to maintain rhythmicity under conditions of stress, perhaps through modulation of clock molecules and circadian output. Of the ~18 known nuclear receptors in Drosophila [36] , only one other, unfulfilled , has been implicated in clock function [37] . However, the mechanism by which it affects the clock is unknown, as is the ligand that activates it. In case of E75, a few natural ligands have been identified such as haem, CO and NO [12] , [13] . REV-ERB also binds to haem and may reset the clock in response to it [38] . It is possible that NO and CO also affect the clock. Future studies of E75 in Drosophila could elucidate mechanisms by which nuclear receptors mediate effects of signalling molecules on circadian clock function. Fly stocks tim -Gal4 27 , (TG 27 ), cry 24 -Gal4, Pdf -Gal4 UAS- E75 RNAi (JF02257 and HMS01530), UAS- EcR B1 ΔC655.F645A , UAS- EcR A-RNAi, UAS- EcR -A, UAS- EcR B2, UAS- EcR -C and E75 Δ51 lines were provided by the Bloomington Stock Center. UAS -E75 II and III were provided by Henry Krause (University of Toronto). UAS- E75 RNAi GD and KK were obtained from the Vienna Drosophila Resource Center. TUG; UAS- Dicer2 and Pdf -Gal4; UAS- Dicer2 lines were from our laboratory. NE30-49-10 EP was an overexpression line generated in our laboratory [16] . The insertion was determined by Inverse PCR in accordance with protocols from the Berkley Drosophila Genome Project. Clk hypo is a Piggybac {WH}f06808 insertion line and was obtained from the Bloomington Stock Center. This element is inserted in the 2nd exon of the Clk gene and our behavioural and molecular analyses suggest that it is a hypomorphic allele of Clk (Kyunghee Koh, personal communication). Locomotor activity assay About 3- to 5-day-old adults were entrained to LD (12:12 h) cycles for 3 days at 25 °C and then were transferred into constant darkness (DD) and their activity was monitored for at least 6–7 days using the Drosophila Activity Monitor system (Trikinetics). Data were obtained and analysed using Clocklab software (ActiMetrics). The periodicity and the strength of the activity:rest rhythm of each fly was determined by visual examination of activity records and χ 2 periodograms and through FFT analysis. Flies displaying distinct single well-defined peaks by χ 2 periodogram and an FFT value of >0.01 were classified as rhythmic individuals and were included for determining the average period and rhythm strength. Individuals with multiple or broad peaks in the periodogram analysis were not counted for period determination, whereas those that showed random activity patterns and no clear peak by periodogram were categorized as arrhythmic. Note that rhythm strength (FFT values) was calculated only for rhythmic individuals. Western blot analysis Western blot assays were performed as previously described [39] . Briefly, 4- to 5-day-old flies were entrained in LD 12:12 h cycles for 3 days. Exactly ten heads were collected on dry ice at indicated time points. For constant dark (DD) experiments, the flies were sampled on the second day. The fly heads were lysed in a homogenization buffer containing 10 mM HEPES (pH 7.5), 100 mM KCl, 1 mM EDTA, 10% glycerol, 0.1% Triton X-100, 5 mM dithiothreitol and 5 mM phenylmethylsulphonyl fluoride along with the phosphatase inhibitors okadaic acid and 1 mM sodium vanadate. A protease inhibitor cocktail (Boehringer) was also added to the buffer according to the manufacturer’s instructions. Homogenates were spun twice for 10 min at 12,000 r.p.m., and the supernatant was transferred to microcentrifuge tubes kept on ice. 15 μl of each sample was run on 4–12% SDS–polyacrylamide mini-gels, and transferred onto nitrocellulose membranes overnight. PER protein was detected with a 1:2,000 dilution of GP anti-PER antibody [40] . This antibody is highly specific to PER with the most intense band detected at approximately 150kDa, the predicted size of Drosophila PER. The other antibodies used in different assays were guinea pig anti-CLK (1:3,000) [41] and mouse anti-HSP70 (1:15,000; Sigma). The western blots were developed by a horseradish peroxidase enzymatic activity-based assay followed by enhanced chemiluminescence (ECL reagent; Thermo Scientific). Blots were stripped using a western blot stripping buffer (Thermo Scientific) and re-probed with a guinea pig anti- CLK antibody (1:3,000). Images were obtained using a Kodak image station or through exposure to X-ray film. These images were analysed by ImageJ software (NIH) for quantification of individual bands. Quantitative real-time PCR Protocols for total RNA isolation and cDNA synthesis have been described previously [39] . Briefly, 3- to 5-day-old adults were entrained to an 12:12 h LD cycle for 3 days at 25 °C and then collected on dry ice at indicated time points on the last day of the LD cycle. Total RNA was isolated using the manufacturer’s protocol (TRIzol; Life Technologies), and cDNAs were synthesized using a high-capacity cDNA reverse Transcription kit (Applied Biosystems; Life technologies). Real-time assays were performed using an ABI prism 7000 with a SYBR Green kit (Applied Biosystems). The oligos used in the assays were Act5C forward (5′- ATGTCACGGACGATTTCACG -3′) and Act5C reverse (5′- CGCGGTTACTCTTTCACCA -3′), per forward (5′- CGTCAATCCATGGTCCCG-3′ ) per reverse (5′- CCTGAAAGACGCGATGGTG -3′), Clk forward (5′- GGATGCCAATGCCTACGAGT -3′), Clk reverse (5′- ACCTACGAAAGTAGCCCACG -3′). Immunohistochemistry Three- to five-day-old adults were entrained to an 12:12 h LD cycle for 3 days at 25 °C and then collected at indicated time points. Adult fly heads were washed in 70% alcohol and brains were dissected in 4% paraformaldehyde (made in PBS) and fixed for ~20 min, washed for 1 h in PBS buffer and followed by overnight incubation with primary antibody (in PBS buffer with 3% normal donkey serum and 0.3% Triton X-100) at 4 °C. Brain samples were washed four to five times with PBS-T (PBS with 0.3% Triton-X) buffer and incubated with Cy3 donkey anti-rabbit (or guinea pig) and fluorescein isothiocyanate or Cy3 donkey anti-rabbit (or mouse) secondary antibodies (Jackson ImmunoResearch Laboratories) for 2 h at room temperature, followed by an additional four to five washes in PBS-T buffer. A Leica TCS SP5 confocal microscope (Leica) was used to obtain the fluorescent images. The primary antibody dilutions used in this assay were as follows: PER, 1:1,000; CLK (GP50), 1:1,000; PDF, 1:1,000; mouse EcR common (Ag10.2) 1:150; mouse EcR-A (15G1a), 1:50. Secondary antibody dilutions were 1:500. The fluorescent intensity of individual cells was measured from confocal images with NIH ImageJ software. The background intensity from the adjacent area was subtracted from these values followed by averaging of the normalized value. Expression constructs For co-transfection studies, the Clk -luc [2] and 4.6 kb per -luc plasmids were generated by inserting genomic DNA upstream of the basal promoter in the luciferase reporter vector pGL3 (Promega). cDNA templates for E75 , kindly provided by Carl Thummel (University of Utah), were used for constructing the expression vectors pMT- E75A and pMT- E75B , which contain full-length E75-RA and E75-RC , respectively, in the Not I and Xba I sites of pMTv5HisA (Invitrogen). All constructs were verified by sequencing. Cell culture luciferase assay For the luciferase reporter-based transcriptional assays, either human embryonic kidney (HEK293T) or Drosophila S2 cells were used. For HEK 293T cell transfection assays, a total of ~10 5 cells were transfected into 24-well plates with the following expression plasmids––CMV- E75 , CMV- pdp1ε , CMV- per -HA, CMV- GFP –together with the reporter Clk - luc and the renilla -luciferase as internal control. Empty pcDNA3.1 vectors were added to control for uniform DNA amounts across transfections using Lipofectamine (LifeTechnologies). A total of 500 ng of DNA was used in each case. Following transfection, the cells were collected after 48 h, lysed and assayed for luciferase activity (Promega). The firefly luciferase measurements were normalized to renilla luciferase activity counts and presented as a ratio. Transfections were conducted as four independent sets and final values were determined by averaging the data obtained from the four replicates. Co-immunoprecipitation assays Mammalian HEK293T cells (~2 × 10 6 ) used were transfected with the following plasmids: pcDNA3- per -HA, pcDNA3.1 E75 , pcDNA3- cry , pcDNA3.1 Gaba-t , using Lipofectamine (Life Technologies) reagent and cells were collected and lysed after 48 h. In all cases, exactly 300 ng of total DNA was transfected. Cell lysates were incubated overnight with primary antibody (HA or PER antibody) and 30 μl of Dynabeads (Life Technologies) in Imunno-precipitation (IP) buffer (10 mM HEPES (pH7.5), 150 mM NaCl, 1 mM EDTA, 1 mM dithiothreitol, 0.3% Triton-X 100, 0.03% SDS and protease inhibitor). The beads were washed extensively in wash buffer, followed by SDS– polyacrylamide gel electrophoresis and western blotting. How to cite this article: Kumar, S. et al . An ecdysone-responsive nuclear receptor regulates circadian rhythms in Drosophila . Nat. Commun. 5:5697 doi: 10.1038/ncomms6697 (2014).